Translation-independent circadian control of the cell cycle in a unicellular photosynthetic eukaryote Circadian rhythms of cell division have been observed in several lineages of eukaryotes, especially photosynthetic unicellular eukaryotes. However, the mechanism underlying the circadian regulation of the cell cycle and the nature of the advantage conferred remain unknown. Here, using the unicellular red alga Cyanidioschyzon merolae , we show that the G1/S regulator RBR-E2F-DP complex links the G1/S transition to circadian rhythms. Time-dependent E2F phosphorylation promotes the G1/S transition during subjective night and this phosphorylation event occurs independently of cell cycle progression, even under continuous dark or when cytosolic translation is inhibited. Constitutive expression of a phospho-mimic of E2F or depletion of RBR unlinks cell cycle progression from circadian rhythms. These transgenic lines are exposed to higher oxidative stress than the wild type. Circadian inhibition of cell cycle progression during the daytime by RBR-E2F-DP pathway likely protects cells from photosynthetic oxidative stress by temporally compartmentalizing photosynthesis and cell cycle progression. The regular 24-h rotation of the earth has led to the emergence, in the course of evolution, of circadian oscillators in virtually all life forms. Circadian rhythms regulate biological processes so as to make them occur at the appropriate time in a specific environment, resulting from daily fluctuations in energy availability [1] , [2] . One of the biological processes controlled by circadian rhythms is the temporal gating of cell division, a phenomenon that has been observed in a wide variety of eukaryotic lineages from unicellular organisms to mammals [3] . The circadian gating of cell division is especially evident in unicellular algae, in which cells divide at night [3] , [4] , [5] , [6] . It is well established that one of the core mechanisms underlying circadian rhythms is the transcription and translation feedback loop (TTFL) of the ‘clock’ transcription factors. The rhythmic expression of the clock gene products in the TTFL regulates the expressional output of other genes in ~24-h cycles [7] . Because the specific transcriptional components differ in different eukaryotic lineages, it is thought that the TTFL has emerged in them independently in the course of evolution [7] . Although the circadian gating of cell division has long been known, especially the regulation of the G1/S transition, the only well-understood underlying mechanism is that of the G2/M transition in mouse liver cells. In the regenerating liver hepatocytes, expression of wee1 (a suppressor of the G2/M transition) is regulated by TTFL so that the G2/M transition is restricted to the morning, when the WEE1 protein level reaches its lowest point [8] . In the case of photosynthetic eukaryotes, a previous transcriptome analysis suggested a model in which the G1/S transition is regulated by the light and time-dependent transcription of G1/S regulators [4] . However, the mechanism of the circadian gating of cell division and the nature of the advantage conferred by such strictly regulated cyclicity in photosynthetic eukaryotes are both still only poorly understood. To address these issues, we have chosen a simple system, the unicellular hot-spring red alga (optimal temperature 42 °C) Cyanidioschyzon merolae . C. merolae possesses an extremely small nuclear genome (16.7 Mb) [9] , which minimizes the set of cell cycle regulators that have to be analysed. Nuclear transformation by homologous recombination has been developed in this alga [10] . In addition, the cell cycle is highly synchronized by a 12-h light/12-h dark (LD) cycle in which cells divide by binary fission during the dark period ( Fig. 1a ); refs 11 , 12 . This is in contrast with many other algae, such as Chlamydomonas reinhardtii, which undergo multiple fission events, thus making it difficult to characterize the progress of the cell cycle. 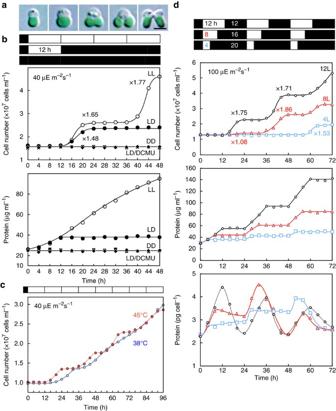Figure 1: The growth-dependent circadian gating of cell division inC. merolae. (a) Microscopic images showing the course of cell division ofC. merolae. The scale bar, 2 μm. (b–d) The changes in the cell number, protein level (per culture and per cell) during synchronous culture. Cells were cultured at 42 °C or otherwise indicated. Cells were entrained by a 12-h light and 12-h dark cycle and then cultured under the same condition (LD), LL, or DD. To block photosynthetic electron flow under the LD condition, DCMU was added to the culture just before the onset of the light period (b). Cells were entrained by a 12-h light and 12-h dark cycle and then cultured under LL at 38 °C or 45 °C (c). After the entrainment, cells were cultured by a 12-, 8- or 4-h light cycle (d). The numbers on the lines indicate the increase in the cell number during 24 h. Two independent experiments showed similar results and results from one experiment are shown. Figure 1: The growth-dependent circadian gating of cell division in C. merolae . ( a ) Microscopic images showing the course of cell division of C. merolae . The scale bar, 2 μm. ( b – d ) The changes in the cell number, protein level (per culture and per cell) during synchronous culture. Cells were cultured at 42 °C or otherwise indicated. Cells were entrained by a 12-h light and 12-h dark cycle and then cultured under the same condition (LD), LL, or DD. To block photosynthetic electron flow under the LD condition, DCMU was added to the culture just before the onset of the light period ( b ). Cells were entrained by a 12-h light and 12-h dark cycle and then cultured under LL at 38 °C or 45 °C ( c ). After the entrainment, cells were cultured by a 12-, 8- or 4-h light cycle ( d ). The numbers on the lines indicate the increase in the cell number during 24 h. Two independent experiments showed similar results and results from one experiment are shown. Full size image By using the unicellular red alga, Cyanidioschyzon merolae , we demonstrate that the timing of the G1/S transition is restricted to early subjective night via a time-dependent phosphorylation of the E2F protein, which does not require protein synthesis (or the TTFL). Further, the uncoupling of cell cycle progression from circadian rhythms substantially exacerbates oxidative stress, suggesting that the temporal sequestration of oxygenic photosynthesis during the daytime and cell cycle progression at night is likely to be critically important to unicellular photosynthetic eukaryotes. Circadian regulation of C. merolae cell division We first asked whether cell division in C. merolae is regulated by circadian rhythms based on the following criteria [1] : the persistence of an ~24-h rhythm under constant conditions, the entrainability of the rhythm (this was already confirmed by the cell division synchronization) and temperature compensation of the rhythm. After entrainment by one round of LD (stationary phase cells were diluted in fresh medium and then entrained), 48% of the cells underwent synchronous cell division during the next dark period under limited light (40 μE m −2 s −1 ) ( Fig. 1b ). When cells were cultured under continuous light (LL) after entrainment, the population of dividing cells increased to 65%. However, 35% did not divide during the first day, and for these cells, the next round of cell division started at the beginning of the next subjective night, even though these cells kept growing continuously under LL (as indicated by the increase in protein content) ( Fig. 1b ). Under high light LL (100 μE m −2 s −1 ), the cell number increased by more than twofold on a given day, but the timing of cell division was biased to subjective night ( Supplementary Fig. 1 ). Thus, cell division is gated so as to predominantly take place during subjective night. When entrained cells were cultured under LL at two different temperatures (45 or 38 °C), the first cell division started at the same time, but subsequently, synchrony was not evident at 38 °C ( Fig. 1c ), most likely because the progression of cell division is delayed at lower temperatures. At this point, the temperature compensation of cell cycle progression is not supported by the findings, but E2F phosphorylation, which is required for G1/S transition, is temperature compensated, as shown below. The relationship between cell growth and cell division Then, we examined the relationship between photosynthetic cell growth and cell division by changing the duration of the light period (4, 8 or 12 h). Under all conditions, the cellular protein level increased only during the light period and the timing of cell division (that is, the increase in the cell number, if it occurred) was restricted to dark period ( Fig. 1d ). Under the 8-h light condition, only a small population (8%) divided on the first day, while most of the cells (86%) divided on the second day ( Fig. 1d ). When cells were cultured under continuous dark (DD) or the photosynthetic electron flow was inhibited by 3-(3,4-dichlorophenyl)-1,1-dimethylurea (DCMU) under LD, no cell division was observed ( Fig. 1b ). Thus, cell division occurs only when the cell has attained a certain threshold (such as a specific cell size or protein content) as the result of photosynthesis, but the decision to divide or not is made only during subjective night. E2F is phosphorylated under control of circadian rhythms This observation led us to investigate two types of cell cycle regulators, one that accumulates in association with the cell growth and another that is regulated by circadian rhythms. A key regulator of the G1/S transition in eukaryotic cells, including eukaryotic algae [4] , [13] , [14] , [15] , is the retinoblastoma (RB) tumour suppressor pathway [16] . RB represses the G1/S transition by binding to the E2F-DP heterodimer, which in turn binds certain specific cis elements of S-phase genes. In animal cells, cyclin D and E accumulate during the G1 phase as the result of cell growth, and the CDK-cyclin D/E phosphorylates RB. This phosphorylation dissociates RB from E2F-DP, which then activates the transcription of the S-phase genes ( Fig. 2a ); ref. 16 . 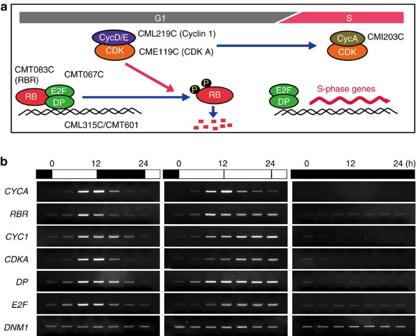Figure 2: The change in the mRNA levels of genes related to G1/S transition. (a) Diagram showing the regulation of the G1/S transition in animal cells. The locus IDs of the corresponding proteins inC. merolaegenome are also indicated. (b)C. merolaecells were entrained by a 12-h light and 12-h dark cycle. Then, the cells were cultured in the same light/dark cycle, under LL or DD condition. The mRNA levels were examined by semi-quantitative RT–PCR analyses.DNM1(CME019C) was used as the quantitative control. Two independent experiments showed similar results and results from one experiment are shown (a–d). Figure 2: The change in the mRNA levels of genes related to G1/S transition. ( a ) Diagram showing the regulation of the G1/S transition in animal cells. The locus IDs of the corresponding proteins in C. merolae genome are also indicated. ( b ) C. merolae cells were entrained by a 12-h light and 12-h dark cycle. Then, the cells were cultured in the same light/dark cycle, under LL or DD condition. The mRNA levels were examined by semi-quantitative RT–PCR analyses. DNM1 (CME019C) was used as the quantitative control. Two independent experiments showed similar results and results from one experiment are shown ( a – d ). Full size image Based on the results of BLAST searches, a previous genome investigation of C. merolae identified genes encoding CDKA, RB-related (RBR), E2F, cyclin A and cyclin B (the top hits were occupied by the respective homologues in other organisms) ( Fig. 2a ). Besides these genes, five other genes encoding cyclin homologues were identified [9] . In a previous transcriptome analysis of C. merolae culture that was synchronized by LD, the mRNA level of only cyclin A, cyclin B and CML219C exhibited an oscillating pattern among the seven cyclin gene families [17] . CML219C (here called cyclin 1) is annotated as cyclin E in the C. merolae genome database [9] , but our new BLASTP search failed to clarify which type of cyclins in other eukaryotes are most closely related to cyclin 1. Based on the pattern of mRNA accumulation under LD [17] , cyclin 1 was examined in this study as a possible functional homologue of cyclin D/E ( Fig. 2a ). First, we looked for a change in the transcript level of G1/S regulators, but no circadian oscillation was found in any of these genes ( Fig. 2b ). The transcript level peaked around the onset of the dark period under LD. However, under LL, only the S-phase cyclin CYCA exhibited an oscillating pattern, peaking at the onset of subjective night, but the others kept accumulating under LL, even though cell division ended at the end of subjective night ( Fig. 1b , and this is also indicated by the reduction of the CYCA transcript level, as shown in Fig. 2b ). Under DD, the transcript level either remained constant or decreased ( Fig. 2b ). Next, we examined changes in the level and phosphorylation state of the G1/S regulating proteins (the specificity of antibodies is shown in Supplementary Fig. 2 ). When cells were cultured under 8-h light LD (a small number on the first day, but most of the population divided on the second day; Fig. 1d ), cyclin A accumulation and RBR phosphorylation were detected only on the second day of division ( Fig. 3a ). Cyclin 1 accumulated during the first light period and the level remained constant during the first dark period without any cell division. Cyclin 1 again accumulated during the second light period and then decreased late in the second dark period after cell division ( Fig. 3a ). Thus, cells on the first day were arrested prior to RBR phosphorylation. Cyclin 1 accumulated during the G1 phase and decreased after the G1/S transition ( Fig. 3a ) in a manner similar to cyclin D/E in animal cells, suggesting that cyclin 1 is likely to be a factor linked to cell growth. 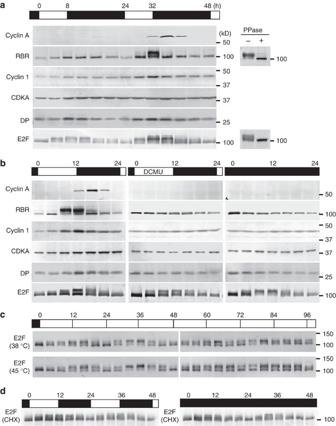Figure 3: E2F is phosphorylated in a time-dependent manner independently of cell cycle progression and protein synthesis. (a,b) Immunoblot analyses showing the change in the levels and phosphorylation states of proteins that are involved in the G1/S transition inC. merolae. Cells were cultured at 42 °C or as otherwise indicated. Cells were entrained by a 12-h light and 12-h dark cycle and then cultured by the 8-h light cycle (a; same asFig. 1c). After the entrainment, cells were cultured under the same conditions or DD (b). Three independent experiments showed similar results and results from one experiment are shown (a,b). The downward band shift of RBR and E2F by the phosphatase treatment indicates that the upper bands correspond to phosphorylated proteins. PPase (+) or (−) indicates that proteins were treated with (+) or without (−) lambda protein phosphatase. DCMU was added to the culture just before the onset of the light period (b; same asFig. 1b). (c) After the entrainment, cells were cultured under LL at 38 °C or 45 °C. (d) After the entrainment, cells were cultured under the same condition or DD. Cycloheximide (CHX) was added to the culture 1 h before the end of the entrainment. Two independent experiments showed similar results and results from one experiment are shown (c,d). Figure 3: E2F is phosphorylated in a time-dependent manner independently of cell cycle progression and protein synthesis. ( a , b ) Immunoblot analyses showing the change in the levels and phosphorylation states of proteins that are involved in the G1/S transition in C. merolae . Cells were cultured at 42 °C or as otherwise indicated. Cells were entrained by a 12-h light and 12-h dark cycle and then cultured by the 8-h light cycle ( a ; same as Fig. 1c ). After the entrainment, cells were cultured under the same conditions or DD ( b ). Three independent experiments showed similar results and results from one experiment are shown ( a , b ). The downward band shift of RBR and E2F by the phosphatase treatment indicates that the upper bands correspond to phosphorylated proteins. PPase (+) or (−) indicates that proteins were treated with (+) or without (−) lambda protein phosphatase. DCMU was added to the culture just before the onset of the light period ( b ; same as Fig. 1b ). ( c ) After the entrainment, cells were cultured under LL at 38 °C or 45 °C. ( d ) After the entrainment, cells were cultured under the same condition or DD. Cycloheximide (CHX) was added to the culture 1 h before the end of the entrainment. Two independent experiments showed similar results and results from one experiment are shown ( c , d ). Full size image In contrast to the other proteins, E2F was phosphorylated and then dephosphorylated on both days in a time-dependent manner, independently of cell cycle progression ( Fig. 3a ). This time-dependent phosphorylation occurred even when photosynthesis and cell division were inhibited, either by DCMU or under DD ( Fig. 3b ). The E2F phosphorylation occurred with a similar timing and the period length was ~24 h at both 38 and 45 °C under LL ( Fig. 3c ), indicating a pattern of temperature compensation. Given these results, it is concluded that E2F phosphorylation is under the control of circadian rhythms. E2F phosphorylation independent of translation In order to determine whether E2F phosphorylation requires a time-dependent expression of a specific kinase or its regulators, or is regulated by the TTFL, we first tested transcription inhibitors (actinomycin D and cordycepin), but these inhibitors were ineffective in C. merolae . Thus, we examined the effect of a translation inhibitor on E2F phosphorylation. As reported previously [18] , cycloheximide inhibited protein synthesis in C. merolae , which was confirmed by there being no increase in the protein level or cell division under LD ( Supplementary Fig. 3 ) compared with the culture without cycloheximide ( Fig. 1b ). Even when cytosolic protein synthesis was inhibited by cycloheximide, the time-dependent E2F phosphorylation was observed ( Fig. 3d ). These results indicate that the time-dependent E2F phosphorylation does not require either time-dependent protein expression or the TTFL. E2F phosphorylation accelerates the G1/S transition The phosphorylation of E2F has been reported only in human cells that have activated G1/S progression [19] . In order to examine the biochemical effect of E2F phosphorylation in C. merolae , the RBR-E2F-DP complex was extracted from synchronized G1 (unphosphorylated E2F) or S-phase (phosphorylated E2F) cells. The pattern of gel filtration indicates that E2F, DP and RBR are included in an ~300 kDa complex in both the G1 and S phases ( Fig. 4a ). Anti-DP and anti-E2F antibodies each co-immunoprecipitated E2F and RBR from both G1 and S-phase cell extracts ( Fig. 4b ). When a partially purified RBR-E2F-DP complex was incubated with the biotin-labelled E2F binding region of PCNA in vitro , E2F and DP were co-precipitated with the DNA by means of avidin beads ( Fig. 4c ). Chromatin immunoprecipitation using the anti-E2F antibody and subsequent quantitative PCR (ChIP–qPCR) analyses showed that E2F binds to the E2F binding region of PCNA and FTSZ2-1 (a chloroplast division gene that is specifically transcribed during the S phase in C. merolae [20] ) loci in both the G1 and S phases in vivo ( Fig. 4d ). Thus, E2F phosphorylation does not change the binding of E2F to DP, RBR and the promoter region of S-phase genes. This observation is consistent with the results in C. reinhardtii , where the RBR-E2F-DP complex is stable throughout the cell cycle [13] , unlike the case in animal cells. 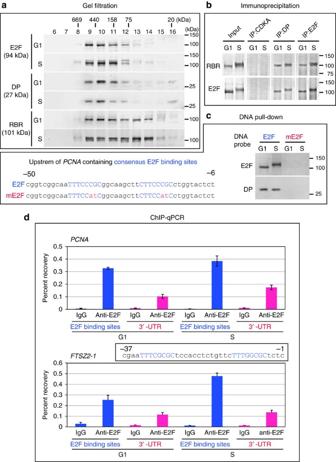Figure 4: The effect of E2F phosphorylation on RBR-E2F-DP complex composition and the binding of E2F to DNA. (a,b) The RBR-E2F-DP complex composition was compared between the G1 phase (unphosphorylated E2F) and the S phase (phosphorylated E2F). The cell extract was separated by gel filtration and E2F, DP and RBR were detected by immunoblotting (a). The cell extracts were probed with anti-CDKA, anti-DP or anti-E2F antibodies and the respective immunoprecipitated fractions were analysed by immunoblotting using anti-RBR and anti-E2F antibodies (b). (c) DNA pull-down was carried out using the E2F enriched fraction by anion-exchange chromatography and an oligonucleotide corresponding to the region upstream of theC. merolae PCNAgene, which contains two E2F binding sequences (DNA probe, E2F) or its mutated version (mE2F). Proteins pulled down with the double-strand probe were analysed by immunoblotting using anti-E2F and anti-DP antibodies. The number above the sequence indicates the position from the transcription start site (+1). (d) ChIP–qPCR analysis of E2F at the E2F binding sequence in G1 or S-phase cells. The E2F-chromatin complex was immunoprecipitated with anti-E2F antibodies. A control reaction was processed in parallel with rabbit IgG. ChIP and input whole-cell lysate DNA samples were quantified by real-time qPCR using primers specific to the E2F binding sequence ofPCNAorFTSZ2-1(the number above the sequence indicates the position from the transcription start site (+1)) and 3′-UTR ofPCNA(~1.8 kbp downstream of the E2F binding sequence) orFTSZ2-1 (~1.7 kbp downstream of the E2F binding sequence). The percent recovery is indicated. Error bars represent the s.d. (n=3). Two independent experiments showed similar results and results from one experiment are shown (a,d). Figure 4: The effect of E2F phosphorylation on RBR-E2F-DP complex composition and the binding of E2F to DNA. ( a , b ) The RBR-E2F-DP complex composition was compared between the G1 phase (unphosphorylated E2F) and the S phase (phosphorylated E2F). The cell extract was separated by gel filtration and E2F, DP and RBR were detected by immunoblotting ( a ). The cell extracts were probed with anti-CDKA, anti-DP or anti-E2F antibodies and the respective immunoprecipitated fractions were analysed by immunoblotting using anti-RBR and anti-E2F antibodies ( b ). ( c ) DNA pull-down was carried out using the E2F enriched fraction by anion-exchange chromatography and an oligonucleotide corresponding to the region upstream of the C. merolae PCNA gene, which contains two E2F binding sequences (DNA probe, E2F) or its mutated version (mE2F). Proteins pulled down with the double-strand probe were analysed by immunoblotting using anti-E2F and anti-DP antibodies. The number above the sequence indicates the position from the transcription start site (+1). ( d ) ChIP–qPCR analysis of E2F at the E2F binding sequence in G1 or S-phase cells. The E2F-chromatin complex was immunoprecipitated with anti-E2F antibodies. A control reaction was processed in parallel with rabbit IgG. ChIP and input whole-cell lysate DNA samples were quantified by real-time qPCR using primers specific to the E2F binding sequence of PCNA or FTSZ2-1 (the number above the sequence indicates the position from the transcription start site (+1)) and 3′-UTR of PCNA (~1.8 kbp downstream of the E2F binding sequence) or FTSZ2- 1 (~1.7 kbp downstream of the E2F binding sequence). The percent recovery is indicated. Error bars represent the s.d. ( n =3). Two independent experiments showed similar results and results from one experiment are shown ( a , d ). Full size image We identified four phosphorylation sites of E2F close to the carboxy terminus by LC-MS/MS analyses ( Fig. 5a ; Supplementary Fig. 4 and Supplementary Table 1 ). In order to examine the effect of E2F phosphorylation on G1/S transition, GFP-tagged, non-mutated, phospho-mutated, phospho-mimic and C-terminal portion (containing the four phosphorylation sites)-truncated versions of GFP-E2F transgenes were transiently transformed into C. merolae , and then the transformants were cultured under dark to arrest the cells in the G1 phase. The transgenes downstream of the heat shock promoter were then expressed by elevating the temperature in the G1 cells under LL ( Fig. 5b ). The level of GFP-E2F expressed from the transgenes was similar to that of E2F translated from the chromosomal E2F locus in a mixture of transformed and untransformed cells ( Fig. 5c ). Because the GFP-positive transformants were ~3% of the total population in these assays, it is estimated that ~30 times an excess of GFP-E2F is present in the GFP-positive transformants. The overexpression of GFP-tagged, non-mutated E2F did not change the percentage of S or M phase cells (that is, containing a dividing or two divided chloroplasts [11] , [12] ) as compared with mock-treated cells ( Fig. 5d ). The overexpression of phospho-mutated or C-terminal truncated E2F decreased the percentage of S/M cells, while overexpression of the phospho-mimic E2F increased S/M cells ( Fig. 5d ). These results suggest that unphosphorylated E2F negatively regulates the G1/S transition, and phosphorylated E2F accelerates the G1/S transition. 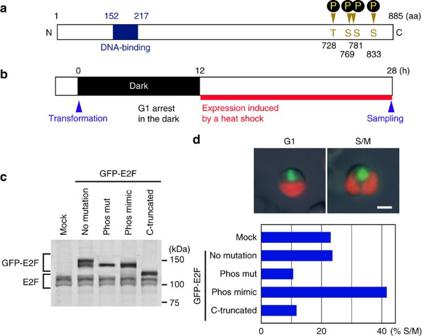Figure 5: E2F phosphorylation accelerates the G1/S transition. (a) The primary structure and positions of the DNA-binding sites (predicted by Pfam) and phosphorylation sites determined by LC-MS/MS analyses. aa, amino acids. (b–d) Transgene encoding GFP-E2F (no mutation), its phospho-mutated (phos mut; the four Ser/Thr were changed to Ala), phospho-mimic (phos mimic; the four Ser/Thr were changed to Asp) or C-terminal portion truncated (C-truncated; containing the four Ser/Thr) variants that were transiently transformed. The cells were arrested in the G1 phase under dark and then expression of the transgene was induced by elevating the temperature (from 38 °C to 48 °C). Cells were harvested 16 h after the induction (b). Expression of GFP-tagged E2F and variants were confirmed by immunoblotting using the anti-E2F antibodies (c). The numbers of GFP-positive transformants with non-dividing single chloroplast (G1 phase) and dividing or divided chloroplasts (S/M phase) were counted (n=100 for all). The fluorescence signal of GFP is green and the autofluorescence of chlorophyll is red. Scale bar, 2 μm (d). Three independent series of transformation showed similar pattern and one representative result is shown (d). Figure 5: E2F phosphorylation accelerates the G1/S transition. ( a ) The primary structure and positions of the DNA-binding sites (predicted by Pfam) and phosphorylation sites determined by LC-MS/MS analyses. aa, amino acids. ( b – d ) Transgene encoding GFP-E2F (no mutation), its phospho-mutated (phos mut; the four Ser/Thr were changed to Ala), phospho-mimic (phos mimic; the four Ser/Thr were changed to Asp) or C-terminal portion truncated (C-truncated; containing the four Ser/Thr) variants that were transiently transformed. The cells were arrested in the G1 phase under dark and then expression of the transgene was induced by elevating the temperature (from 38 °C to 48 °C). Cells were harvested 16 h after the induction ( b ). Expression of GFP-tagged E2F and variants were confirmed by immunoblotting using the anti-E2F antibodies ( c ). The numbers of GFP-positive transformants with non-dividing single chloroplast (G1 phase) and dividing or divided chloroplasts (S/M phase) were counted ( n =100 for all). The fluorescence signal of GFP is green and the autofluorescence of chlorophyll is red. Scale bar, 2 μm ( d ). Three independent series of transformation showed similar pattern and one representative result is shown ( d ). Full size image E2F phosphorylation links the G1/S to circadian rhythms In order to examine the role of the time-dependent E2F phosphorylation in the circadian gating of cell division, we tried to knockout the E2F locus. Despite several efforts, we were unable to obtain a knockout colony, suggesting that E2F is essential for the proliferation of C. merolae . The C. merolae genome encodes two copies of the DP protein ( Fig. 2a ; 98% identical in amino-acid sequence) in distinct chromosomes and, at present, only one transformation marker is available. Thus, we gave up the effort to knockout the DP loci. Because of these limitations, we prepared a strain that constitutively expresses a GFP-phospho-mimic of E2F ( E2F -p) from a genomic-neutral locus. (A phospho-mutated version was not prepared because its transient expression suppressed the G1/S transition ( Fig. 5 )). In addition, we succeeded in obtaining an RBR knockout strain (Δ RBR ) ( Fig. 6a ). 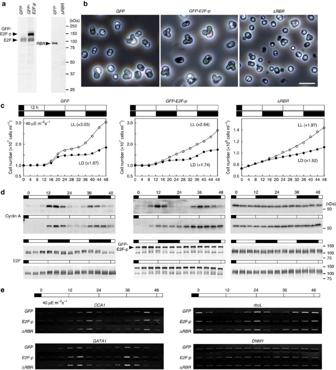Figure 6: Constitutive expression of phospho-mimic E2F or depletion of RBR uncouples cell cycle progression from circadian rhythms. (a) Immunoblot analyses showing constitutive expression of phospho-mimic-E2F (GFP-E2F-p; left) and depletion of RBR (ΔRBR; right). For comparison, cells overexpressing GFP (GFP) were used. All of the three strains are transformants based on the same background (C. merolaeM4 that has a mutation in theURAgene). (b) Phase-contrast images of GFP overexpresser (GFP), GFP-tagged phospho-mimic-E2F overexpresser (GFP-E2F-p) andRBRknockout (ΔRBR) cells. (c,d) The changes in the cell number (c), Cyclin A level and E2F phosphorylation level (d) under 12-h light/12-h dark (LD) or LL. Cells were entrained by a 12-h light and 12-h dark cycle and then cultured under LD or LL. (e) Semi-quantitative RT–PCR analyses showing the expression patterns ofCCA1(CMK043C),GATA1(CMR493C) andrbcL(CMV013C) under LL after the entrainment.DNM1(CME019C) was used as the quantitative control. Two independent transgenic lines (for bothGFP-E2F-pand ΔRBR) showed similar results and results from single lines are shown (a–e). Figure 6: Constitutive expression of phospho-mimic E2F or depletion of RBR uncouples cell cycle progression from circadian rhythms. ( a ) Immunoblot analyses showing constitutive expression of phospho-mimic-E2F ( GFP-E2F-p ; left) and depletion of RBR (Δ RBR ; right). For comparison, cells overexpressing GFP ( GFP ) were used. All of the three strains are transformants based on the same background ( C. merolae M4 that has a mutation in the URA gene). ( b ) Phase-contrast images of GFP overexpresser ( GFP ), GFP-tagged phospho-mimic-E2F overexpresser ( GFP-E2F-p ) and RBR knockout (Δ RBR ) cells. ( c , d ) The changes in the cell number ( c ), Cyclin A level and E2F phosphorylation level ( d ) under 12-h light/12-h dark (LD) or LL. Cells were entrained by a 12-h light and 12-h dark cycle and then cultured under LD or LL. ( e ) Semi-quantitative RT–PCR analyses showing the expression patterns of CCA1 (CMK043C), GATA1 (CMR493C) and rbcL (CMV013C) under LL after the entrainment. DNM1 (CME019C) was used as the quantitative control. Two independent transgenic lines (for both GFP-E2F-p and Δ RBR ) showed similar results and results from single lines are shown ( a – e ). Full size image Δ RBR, but not E2F -p, exhibits a small cell phenotype (one-eighth of the wild type in volume on average) ( Fig. 6b ). This result is consistent with a previous study, which showed that a C. reinhardtii mat3 mutant exhibits a small cell phenotype and that MAT3 encodes the RBR protein [21] . The cell division of Δ RBR was not synchronized under LD or LL, even after entrainment ( Fig. 6c,d ; indicated by the constitutive increase of the cell number and the presence of cyclin A-expressing S-phase cells). E2F -p cell division was not synchronized under LL, but it was synchronized under LD. Under LD, the E2F -p cells entered into the S phase (as indicated by cyclin A expression) earlier than the control strain (the GFP overexpresser) ( Fig. 6c,d ). Thus, in E2F -p, entrance into the S phase was not restricted to subjective nights under both LL and LD. ( Fig. 6c,d ). The partial synchronization of E2F -p cell division under LD is probably because the cells enter into the S phase immediately when the cell has grown to a certain threshold size and, during the dark period, cells no longer grow and thus entry into the S phase ceases. In Δ RBR , the circadian E2F phosphorylation pattern, but not E2F phosphorylation itself, was also impaired in contrast to E2F -p ( Fig. 6d ). This result suggests that the presence of RBR in the RBR-E2F-DP complex is required for the circadian regulation of E2F phosphorylation, but the reason is unclear at present. Although cell cycle progression was not synchronized in E2F -p under LL, or Δ RBR under either LD or LL, both lines exhibited an oscillating expression pattern of CCA1 (a dawn-phased myb-like transcription factor of the TTFL) [1] , GATA1 (a circadian-regulated transcription factor related to nitrogen metabolism) [22] and chloroplast-encoded rbcL , all in a manner similar to the wild type ( Fig. 6e ) under LL after entrainment. These results suggest that the circadian regulation of various cellular phenomena other than cell cycle progression is still working in E2F -p and Δ RBR, and that cell cycle progression is uncoupled from circadian rhythms in these transgenic lines. Noncircadian cell cycle increases oxidative stress Circadian rhythms are believed to maximize fitness by enabling organisms to coordinate with the changes that occur in the 24-h environmental cycle by a temporary reorganization of a variety of cellular physiological processes [1] . Although circadian regulation of the cell cycle is evident in many eukaryotes, especially in photosynthetic organisms [3] , the specific survival benefits derived from circadian regulation of cell cycle have not yet been determined. The growth rate of E2F -p ( × 2.64 per 2 days under LL; × 1.74 per 2 days under LD) and Δ RBR ( × 1.97 per 2 days under LL; × 1.52 per 2 days under LD) was less than that of the control strain (the GFP overexpressor) ( × 3.03 per 2 days under LL; × 1.97 per 2 days under LD) ( Fig. 6c ). In addition, the expression of oxidative stress markers such as catalase (an H 2 O 2 scavenger), RAD51 (involved in DNA repair) [23] and 8-oxoguanine-DNA-glycosylase (responsible for the excision of 8-oxoguanine, a mutagenic base byproduct by reactive oxygen species, from DNA) was upregulated in E2F -p and Δ RBR compared with the control strain ( Fig. 7 ). These results indicate that E2F -p and Δ RBR are exposed to a higher level of oxidative stress than the wild type. 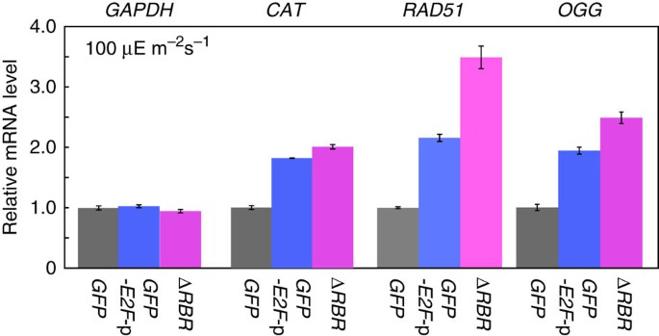Figure 7: The uncoupling of cell cycle progression from circadian rhythms increases oxidative stress. Quantitative RT–PCR analyses showing the expression levels of glyceraldehyde 3-phosphate dehydrogenase (GAPDH; CMM167C) catalase (CAT; CMK043C),RAD51(CMR493C) and 8-oxoguanine-DNA-glycosylase (OGG; CML249C) in the GFP overexpresser (GFP), GFP-tagged phospho-mimic-E2F overexpresser (GFP-E2F-p) andRBRknockout (ΔRBR) cells.EF-1awas used as the internal control. Cells were cultured non-synchronously for 2 days under LL without entrainment. Two independent experiments showed similar results and results from one experiment are shown. Figure 7: The uncoupling of cell cycle progression from circadian rhythms increases oxidative stress. Quantitative RT–PCR analyses showing the expression levels of glyceraldehyde 3-phosphate dehydrogenase ( GAPDH ; CMM167C) catalase ( CAT ; CMK043C), RAD51 (CMR493C) and 8-oxoguanine-DNA-glycosylase ( OGG ; CML249C) in the GFP overexpresser ( GFP ), GFP-tagged phospho-mimic-E2F overexpresser ( GFP-E2F-p ) and RBR knockout (Δ RBR ) cells. EF-1a was used as the internal control. Cells were cultured non-synchronously for 2 days under LL without entrainment. Two independent experiments showed similar results and results from one experiment are shown. Full size image It has been shown using C. merolae that (1) there is a circadian rhythm involved in E2F phosphorylation, (2) this circadian rhythm gates the G1/S transition when a cell has grown over a certain threshold and (3) constitutive phosphorylation of E2F or depletion of RBR unlinks cell cycle progression from circadian rhythms. These findings suggest that the RBR-E2F-DP pathway links the G1/S transition to circadian rhythms through E2F phosphorylation so that the cell cycle does not progress during the daytime ( Fig. 8 ). 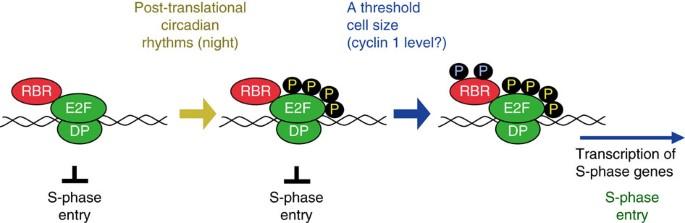Figure 8: Diagram showing the circadian regulation of the G1/S transition by the RBR-E2F-DP complex. E2F-DP binds theciselement of S-phase genes throughout the cell cycle. RBR inhibits the transcriptional activity of E2F-DP. The G1/S transition is gated by the circadian rhythm of E2F phosphorylation, peaking during early subjective night. This phosphorylation is probably dependent on the circadian rhythmic activity of E2F phosphorylation, but does not require the time-dependent expression of kinases or their regulators. The E2F phosphorylation gives ‘permission’ for RBR to be phosphorylated. RBR is phosphorylated only when the cell has grown beyond a certain size threshold. As in the case of cyclin D/E in animal cells, the cyclin 1 level is likely monitoring the cell size. RBR phosphorylation inactivates RBR, thereby enabling E2F-DP to transcribe S-phase genes. Figure 8: Diagram showing the circadian regulation of the G1/S transition by the RBR-E2F-DP complex. E2F-DP binds the cis element of S-phase genes throughout the cell cycle. RBR inhibits the transcriptional activity of E2F-DP. The G1/S transition is gated by the circadian rhythm of E2F phosphorylation, peaking during early subjective night. This phosphorylation is probably dependent on the circadian rhythmic activity of E2F phosphorylation, but does not require the time-dependent expression of kinases or their regulators. The E2F phosphorylation gives ‘permission’ for RBR to be phosphorylated. RBR is phosphorylated only when the cell has grown beyond a certain size threshold. As in the case of cyclin D/E in animal cells, the cyclin 1 level is likely monitoring the cell size. RBR phosphorylation inactivates RBR, thereby enabling E2F-DP to transcribe S-phase genes. Full size image As shown in green algae [4] , [13] , [14] , [15] , the Δ RBR C. merolae cell enters into the S phase even before growing to a certain threshold size ( Fig. 6 ). In contrast, E2F -p cells enter into the S phase only when cells have grown beyond this size threshold ( Fig. 6 ). In both the Δ RBR and E2F -p cells, the G1/S transition is not restricted to early subjective night as it is in wild-type cells ( Fig. 6 ). Given these results, the following scheme of G1/S transition is suggested. Circadian phosphorylation of E2F (peaking during early subjective night; in E2F -p, anytime) gives ‘permission’ for RBR to be phosphorylated; RBR is phosphorylated (inactivated) so as to allow the cell to enter into the S phase only when the cell has grown beyond a certain size threshold ( Fig. 8 ). Thus, the RBR-E2F-DP complex, as a suppressor of the G1/S transition in the unphosphorylated state, functions as a processor, the inputs of which comprise both timing (recognized as E2F phosphorylation) and cell size (recognized as RBR phosphorylation) and the output is the G1/S transition (the transcription of S-phase genes). At this point, how E2F phosphorylation is itself mechanistically linked to circadian rhythms remains unclear. Given that the time-dependent E2F phosphorylation was observed in the absence of light or translation ( Fig. 2c,e ), this phosphorylation does not require time-dependent transcription/translation of kinases or their regulators and is not under the control of the TTFL. It might be dependent on the circadian oscillation of an as-yet-unknown E2F kinase activity under the control of the metabolic/redox circadian cycle, which was recently shown to oscillate in the absence of the TTFL [24] , [25] . In animal cells, the cyclin D/E levels are believed to be a cell size monitor, and in this regard [26] , the cyclin 1 level is likely to monitor the cell size in C. merolae, because the level increases only when the cell is growing during the light period and decreases after cell division ( Fig. 3a ). In the green alga Chlamydomonas reinhardtii , a dp1 -null allele and e2f alleles, in which the genomic region encoding C-terminal portion of E2F is deleted (the amino-terminal DNA-binding domain is intact), were identified as suppressers of the small cell phenotype of the mat3 ( rbr ) mutant [14] . Although the relationship between circadian rhythms and cell cycle progression has not been characterized in these mutants, cell division was shown to be synchronized under LD, but the cells entered the S/M phases 2–4 h earlier than the wild-type cells [14] , similar to the C. merolae E2F -p cells. Based on this similarity, it is possible that the RBR-E2F-DP pathway also links the G1/S transition to circadian rhythms in green algae. Regarding E2F phosphorylation, the top hits of a BLASTP search using C. merolae E2F as a query were occupied by E2F proteins of green algae and land plants. However, the C-terminal portion of E2F, which includes the four phosphorylation sites in the case of C. merolae, is not conserved among photosynthetic eukaryotes, and it is also not conserved among other eukaryotic lineages in terms of the primary structure. Thus, further studies are required to investigate the involvement of E2F phosphorylation in the circadian control of the G1/S transition in green algae and other eukaryotic lineages. In this study, it was shown that E2F -p and Δ RBR are exposed to a higher level of oxidative stress than the wild type ( Fig. 7 ). Circadian rhythms in photosynthetic eukaryotes temporally segregate the physiological pathways in which photosynthetic activity peaks during subjective daytime [27] . Thus, the temporal sequestration of cell cycle progression apart from photosynthesis, which intrinsically produces ROS [23] , is likely to be important for unicellular photosynthetic eukaryotes in order to help them cope with photosynthetic oxidative stress. However, circadian regulation of cell division is not evident in multicellular land plants. In terms of cell cycle progression and photosynthesis, seed plants appear to have evolved a different strategy that depends on plastid differentiation. In seed plants, cell division is restricted to meristematic tissues, and proplastids in the shoot apical meristem are devoid of colour and nonphotosynthetic [28] . Proplastids differentiate into photosynthetic chloroplasts during the development of leaf cells that expand without any cell division (but with endoreduplication) [28] . Thus, photosynthesis and cell division are spatially separated by cell type differentiation in seed plants. In budding yeast under nutrient-limited conditions, the cells rhythmically alternate between glycolysis (reductive phase) and respiration (oxidative phase) over a cycle of 4 to 5 h, and DNA replication is restricted to the reductive phase. It was shown that this temporal restriction of the S phase reduces the occurrence of mutations in the genome [29] . Thus, the temporal separation of ROS-producing photosynthesis and respiration from cell cycle progression is likely to be critical for eukaryotic cells. Culture conditions C. merolae 10D and its derivatives were grown in 2 × Allen’s medium [11] . For the synchronization of C. merolae , the cells in stationary culture (~5 × 10 8 cells per ml at 30 °C) were subcultured to <1 × 10 7 cells per ml −1 in 500 ml flat bottles and subjected to a 12-h light/12-h dark cycle (100 μE m −2 s −1 ) at 42 °C, unless otherwise indicated, under aeration with ordinary air (3 l min −1 ). For DCMU treatment, a 1/1,000 volume of 10 mM DCMU stock solution in ethanol was added just before the onset of the light period. For cycloheximide treatment, a 1/10,000 volume of 10 mg ml −1 cycloheximide stock solution in distilled water was added 1 h before the end of the 12-h light/12-h dark entrainment. The cell number was counted with a Coulter Counter (Z2, Beckman Coulter). For the protein assay, cells were harvested from 1 ml of culture by centrifugation at 800 g for 10 min (0.01% Tween-20 was added just before centrifugation to prevent adsorption of the cells to the tube). The cell pellet was resuspended in 100 μl of 20 mM Tris–HCl, pH 7.5, 8 M urea and 0.1% NP-40. Protein content in the cell lysate was determined by Bradford assay (Protein assay; Bio-Rad). Semi-quantitative and quantitative RT–PCR Cells were harvested from 5 ml culture by centrifugation and stored at −80 °C until RNA extraction. Total RNA was extracted using an RNeasy Plant Mini Kit (Qiagen). After DNaseI treatment, cDNA was synthesized from the RNA using oligo(dT) (15 nucleotides) primer with ThermoScript RT (Life Technologies). For semi-quantitative RT–PCR, the PCR reactions were performed using the primers listed in Supplementary Table 2 . After electrophoresis, amplified cDNA was stained with GelRed Nucleic Acid Gel Stain (Biotium). qPCR amplification was performed using Power SYBR Green PCR Master Mix (Applied Biosystems) in a real-time PCR system (StepOne Plus; Applied Biosystems) using the primers listed in Supplementary Table 2 . Preparation of antibodies and immunoblot analyses The antibodies against C. merolae cyclin A (CMI203C), RBR (CMT083C), cyclin 1 (CML219C), DP (CML315C) and E2F (CMT067C) were raised in rabbits using the respective recombinant proteins. The cDNA sequence encoding the full length or a partial fragment of the respective protein was amplified by PCR using the primers listed in Supplementary Table 1 . These PCR products were cloned into a pET100 expression vector (Life Technologies) and 6xHis fusion polypeptides were expressed in Rosetta (DE3) Escherichia coli cells, purified using a HisTrap HP column (GE Healthcare) and used as antigens. Antibodies were affinity purified from the respective antisera by using respective recombinant polypeptides coupled to a HiTrap NHS-activated HP column (GE Healthcare). To detect C. merolae CDKA (CME119C), anti-PSTAIRE (#541330, Calbiochem) rabbit polyclonal antibody was used. Cells were harvested from 5 to 15 ml of culture by centrifugation and stored at −80 °C until immunoblot analyses. Cells were suspended in the SDS–PAGE sample buffer (50 mM Tris, pH 6.8, 6% 2-mercaptoethanol, 2% sodium dodecyl sulphate, 10% glycerol), separated on 10% SDS-polyacrylamide gels and transferred onto polyvinylidene difluoride membranes (Immobilon; Millipore). For immunoblotting, antibodies against cyclin A (1:2,000), RBR (1:10,000), cyclin 1 (1:5,000), DP (1:2,000), E2F (1:2,000) and CDKA (1: 20,000) were diluted as indicated. The primary antibodies were detected by horseradish peroxidase-conjugated goat anti-rabbit antibody diluted to 1:10,000. The signal was detected by ECL Plus Western Blotting Detection Reagents (GE Healthcare). We confirmed that the signal was not saturated by a comparison of the images from the longer and shorter exposure time periods. For phosphatase treatment, cells were sonicated (Cosmobio, Bioruptor UCW-310, 310 W, 10 cycles of 30 s with a 30 s rest period) with phosphatase buffer (50 mM HEPES-KOH, pH 7.5, 100 mM NaCl, 2 mM DTT, Complete Mini, protease inhibitor mixture (Roche). The cell lysate was incubated with the phosphatase buffer containing 2 mM MnCl 2 and 4,000 units per ml lambda protein phosphatase (New England Biolabs) at 30 °C for 1 h. Gel Filtration and Immunoprecipitation Synchronized cells were harvested by centrifugation at 4 °C from 250 ml of culture. The pellets were resuspended in 3 ml of the cell lysis buffer (20 mM HEPES-KOH, pH 8.0, 1 mM MgCl 2 , 0.2 mM EDTA, 0.5 mM DTT, 0.01% Triton X-100, Complete Mini, protease inhibitor mixture) supplemented with 0.2 M NaCl and the phosphatase inhibitor mixture (25 mM NaF, 2.5 mM Na 3 VO 4 , 5 mM Na 4 P 2 O 7 , 5 mM ß-glycerophosphate) and then broken by sonication. The cell lysate was centrifuged at 100,000 g for 1 h at 4 °C and the supernatant fraction (adjusted to 2 mg protein per ml) was fractionated in the cell lysis buffer using the HiPrep 16/60 Sephacryl S-300HR (GE Healthcare) at a flow rate of 0.5 ml per min. Proteins in the fractions were precipitated by trichloroacetic acid and analysed by immunoblotting. The supernatant fraction of the ultracentrifugation (200 μl, 2 mg protein per ml) and 2 μg of the antibodies were incubated at 4 °C for 1 h. The mixture was then incubated with 50 μl of Dynabeads M-280 Sheep anti-Rabbit IgG (Life Technologies) at 4 °C for 1 h then washed with the cell lysis buffer three times. The washed beads were incubated with 50 μl of the SDS–PAGE sample buffer at 96 °C for 20 min. The extracted proteins in the sample buffer were analysed by immunoblot analyses. DNA pull-down assay The supernatant fraction of the ultracentrifugation (5 ml, 2 mg protein per ml) prepared as above without NaCl in the buffer was applied to 1 ml HiTrap Q HP (GE Healthcare). The column was washed with 5 ml of the cell lysis buffer without NaCl and then the buffer with 200 mM NaCl. Bound proteins, including the RBR-E2F-DP complex, were eluted with the cell lysis buffer with 3 ml of 500 mM NaCl and dialyzed against the cell lysis buffer with 50 mM NaCl. The DNA oligonucleotide 5′-CGGTCGGCAA TTTCCCGC GGCAAGCTT CTTCCCGC CTGGTACTCT-3′ that corresponds to the upstream sequence of C. merolae PCNA (CMS101C) and has two consensus E2F binding sites (underlined) and a mutated version 5′-CGGTCGGCAA TTTCCatC GGCAAGCTT CTTCCatC CTGGTACTCT-3′ (small letters) were each end-labelled with biotin and annealed to complementary DNA oligonucleotides to generate double-stranded probes for the DNA pull-down assay. Two-hundred microliters of the dialyzed fraction (~2 mg protein per ml) were incubated with 1 μg of biotinylated double-strand DNA probe and 10 μg of salmon DNA for 1 h at 4 °C. The mixture was incubated with 50 μl of Dynabeads M-280 Streptavidin (Life Technologies) for 1 h at 4 °C. After washing with the cell lysis buffer containing 50 mM NaCl, proteins bound to DNA probes were extracted by 50 μl of the SDS–PAGE sample buffer. The extracted proteins in the sample buffer were analysed by immunoblot analyses. ChIP–qPCR analysis ChIP–qPCR analysis was performed as previously described [30] except for using the StepOne Plus Real Time System (Applied Biosystems). In brief, synchronized cells were fixed with 1% formaldehyde, treated with micrococcal nuclease and then lysed. Immunoprecipitation was performed using the E2F antibody or rabbit immunoglobulin G (IgG; Sigma-Aldrich). Quantitative real-time PCR was performed with the primers listed in Supplementary Table 2 . Identification of the E2F phosphorylation sites Phosphorylation sites of E2F were identified by LC-MS/MS. The 500 mM NaCl eluate of HiTrap Q HP (for the DNA pull-down assay, as described above) was resolved by SDS–PAGE. A 90–110 kDa region was excised from the gel, digested with trypsin, AspN, Glu-C or Lys-C and then applied to LC-MS/MS. Database searches were performed using the software programme MASCOT (Matrix Science, MA, USA). Only peptides that were identified with a Mascot Ion Score more than 30 were evaluated for both regular and phosphopeptides. For phosphopeptides, the peaks of the neutral loss of H 3 PO 4 were also identified to confirm the phosphorylation. Transient expression of GFP-E2F and its variants To express an N-terminal GFP fusion of E2F that is regulated by the C. merolae HSP20 promoter, we made a construct including the HSP20 promoter, GFP , E2F and nos terminator. The HSP20 promoter was amplified by the primers Xba I_HSP20pro_F and Bgl II_HSP20pro_R, GFP was amplified by Bam HI_GFP_inf_F and Not I_GFP_inf_R, E2F orf was amplified by Not I_E2F_inf_F and Not I_E2F_inf_R. These PCR products were cloned into a pTH2 vector [31] containing the nos terminator, by ligation and In-Fusion Cloning (Takara Bio). The E2F C-terminal portion truncated version (the start codon to the endogenous Bam HI site) was created by amplification of E2F by Not I_E2F_inf_F and Bam HI_NotI_E2F_R. The phospho-mutated (the four serine/threonine sites were changed to alanine) version was created by replacing the sequence encoding C-terminal portion of E2F by synthetic DNA, 5′- ggatcc agagggccacactGCGcctccgaggtacaagcacctgcatgccgttggcgaggatgctgtcgatgatttt catggcgaagtgctgaatcttcgacgtcaacaggaacgcggagaaacgctgcacccggg aacggtgGCTccgggcgggacgcttaaacttcggcgagcatcaGCAccgtacgcgtcgccgctcatcg acggcgtgcaacgcttctcgccatttcgacgaggtgctgttggcgctgggcttcatttagattacg agcttgacggtagctttagtggtatgttggcttgtgttagcggaggagcgctcactcgaag cccgGCGccgcccttgcttcaggatctggctgttgagagccttctcctggaccatactcgg gatagagctatctgtggcaacagcagcagcggtggcgttggcg gcagcaacctcatggatctgttcatctccacagagccggattttgaacgctcgctgagc-3 ′ (the Bam HI site is underlined and the mutated sites are capitalized). The phospho-mimic (the four serine/threonine sites were changed to aspartic acid) version was created by replacing the sequence encoding C-terminal portion of E2F by synthetic DNA. 5′- ggatcc agagggccacactGATcctccgaggtacaagcacctgcatgccgttggcgaggatgctgtcgatgatttt catggcgaagtgctgaatcttcgacgtcaacaggaacgcggagaaacgctgcacccgggaac ggtgGAtccgggcgggacgcttaaacttcggcgagcatcaGATccgtacgcgtcgccgctcatcgac ggcgtgcaacgcttctcgccatttcgacgaggtgctgttggcgctgggcttcatttagattacgagcttgacggta gctttagtggtatgttggcttgtgttagcggaggagcgctcactcgaagcccgGATccgcccttgcttcaggatctggctgttgag agccttctcctggaccatactcgggatagagctatctgtggcaacagcagcagcggtgg cgttggcggcagcaacctcatggatctgttcatctccacagagccggattttgaacgctcgctgagc- 3′ (the Bam HI site is underlined and the mutated sites are capitalized). The resultant plasmids were transiently transformed into C. merolae wild-type cells, as previously described [32] . To express the transgenes in G1-phase cells, cells were arrested in G1 under dark for 12 h before induction of the expression by transferring the cells into 48 °C from 38 °C. The details on the general use of this inducible expression system by using the HSP20 promoter will be published elsewhere, but the information is available upon request. RBR knockout and the phospho-mimic-E2F overexpresser To inactivate the RBR gene, the RBR locus was replaced by the C. merolae URA gene by homologous recombination. The RBR genomic region was amplified with the primers RBR _KO_F1 and RBR _KO_R1. The amplified DNA was cloned into the vector pGEM-T Easy (Promega). The 3′ portion, vector and 5′ portion of RBR were amplified with the primers RBR _KO_F2 and RBR _KO_R2 and then the URA gene amplified with URA_F and URA_R was inserted by In-Fusion Cloning. The RBR genomic region with the URA insert was cut out from the vector by Not I and was transformed into C. merolae M4, a derivative of C. merolae 10D, which has a mutation in the URA gene [10] . Transformation and selection of the gene knockouts were performed as described [33] . To produce the GFP-phospho-mimic E2F overexpresser, the orf of GFP -phospho-mimic E2F (used for transient expression above) was amplified with primers G-E2F -p_F1 and G-E2F -p_R1. The amplified product was inserted into a pD184-O250- EGFP-URA Cm-Cm vector [34] containing the constitutive APCC promoter for expression of the inserted gene and the URA gene between two C. merolae genomic sequences for homologous recombination with a genomic locus (between CMD184C and CMD185C ). The DNA sequence for homologous recombination was amplified with the primers D184F and D184R and transformed into C. merolae M4 as described [34] . How to cite this article: Miyagishima, S.-y. et al. Translation-independent circadian control of the cell cycle in a unicellular photosynthetic eukaryote. Nat. Commun. 5:3807 doi: 10.1038/ncomms4807 (2014).